Pharmacological correction of obesity-induced autophagy arrest using calcium channel blockers Autophagy deregulation during obesity contributes to the pathogenesis of diverse metabolic disorders. However, without understanding the molecular mechanism of obesity interference in autophagy, development of therapeutic strategies for correcting such defects in obese individuals is challenging. Here we show that a chronic increase of the cytosolic calcium concentration in hepatocytes during obesity and lipotoxicity attenuates autophagic flux by preventing the fusion between autophagosomes and lysosomes. As a pharmacological approach to restore cytosolic calcium homeostasis in vivo , we administered the clinically approved calcium channel blocker verapamil to obese mice. Such treatment successfully increases autophagosome–lysosome fusion in liver, preventing accumulation of protein inclusions and lipid droplets and suppressing inflammation and insulin resistance. As calcium channel blockers have been safely used in clinics for the treatment of hypertension for more than 30 years, our results suggest they may be a safe therapeutic option for restoring autophagic flux and treating metabolic pathologies in obese patients. Macroautophagy (hereafter referred to as autophagy) is a highly conserved bulk degradation system that is responsible for degrading long-lived cytoplasmic proteins, protein aggregates, lipid droplets and damaged or excess organelles. An isolation membrane or phagophore expands and encloses a portion of cytosol to form a double-membrane vesicular structure called autophagosome. An autophagosome then fuses with a lysosome to degrade its sequestered contents by lysosomal enzymes [1] , [2] . Autophagy has been shown to be important for regulating physiological functions such as protein turnover, lipid droplet digestion and organelle quality control [3] , [4] . Defects in autophagy are found in various pathological conditions including cancer, obesity, steatosis, insulin resistance and neurodegenerative diseases [5] , [6] , [7] . Lipotoxicity occurs when excessive free fatty acids become accumulated in non-adipose tissues or cells such as hepatocytes and pancreatic cells, contributing to pathogenesis of obesity, diabetes and their related metabolic disorders [8] , [9] , [10] . Saturated fatty acids (SFA) are known to cause more lipotoxic effects that can lead to steatosis and cell apoptosis than unsaturated fatty acids (UFA) [11] , [12] . SFA can cause endoplasmic reticulum (ER) stress and c-Jun N-terminal kinases (JNK) activation as well by increasing ER membrane rigidity [12] , [13] . The reduction in ER membrane fluidity results in inhibition of sarco-ER calcium pump (SERCA), which subsequently elevates cytosolic calcium level. Thapsigargin (Tg), a pharmacological agent known to inhibit SERCA, can provoke autophagosome accumulation by specifically inhibiting autophagy at the autophagosome–lysosome fusion step [14] , [15] . Obesity and SFA also induce autophagosome accumulation; however, it has been elusive whether this is due to increased autophagosome formation or decreased autophagosome degradation [16] , [17] , [18] , [19] , [20] , [21] , [22] . p62, also known as sequestosome-1, is a scaffold protein that plays multiple roles in signalling pathways [23] . In autophagy, p62 is important for targeting ubiquitinated proteins to be transported to the autophagic machinery for their clearance in lysosomes [23] . However, association of ubiquitinated proteins with p62 is not sufficient for autophagic removal, and for this reason, p62-associated ubiquitinated protein aggregates are often identified in diseased tissues of liver dysfunction, neurodegeneration and cancer [24] . Because genetic deletion of p62 actually alleviates the detrimental consequences of autophagy defects in many pathological contexts [25] , [26] , [27] , accumulation of p62 has been considered harmful rather than beneficial for cells. Notably, obesity induces excessive accumulation of p62 and ubiquitinated proteins inside liver, which is an early marker of non-alcoholic steatohepatitis (NASH) pathologies [24] , [28] , [29] . These findings collectively indicate that obesity causes defective autophagy [20] , [22] , [29] . To examine how lipotoxicity, thus obesity, affects autophagy, we developed an in vitro system where cultured human hepatoma (HepG2) cells exhibit prominent accumulation of p62 and ubiquitinated proteins in insoluble inclusion bodies on SFA treatment. As protein inclusion formation was revealed to be a consequence of arrested autophagic flux, we were interested in finding appropriate pharmacological methods that could reverse the effect of SFA on autophagy and protein homeostasis. We found in this study that calcium channel blockers, which can decrease cytosolic calcium level in SFA-treated cells, can restore the autophagic flux and prevent metabolic pathologies associated with autophagy defects. Our results also show that a chronic increase in cytosolic calcium concentration and subsequent inhibition of autophagosome–lysosome fusion are the causes of autophagy arrest during SFA treatment and obesity. Therefore, our study provides an explanation on how obesity-associated lipotoxicity interferes with autophagy overall and suggests a new therapeutic strategy for the obesity-associated autophagy defects. SFA induces p62- and ubiquitin-positive inclusions During obesity and NASH, excessive fat accumulation inside hepatocytes can provoke formation of protein inclusions consisting of p62 and ubiquitinated proteins [24] , [28] . Since the process of inclusion body formation was yet to be explored, we devised an in vitro system that made it possible to examine the effect of lipids on protein aggregation. We found that, in response to palmitic acid (PA, 500 μM), which is a long-chain SFA that becomes highly elevated in sera of obese individuals, human HepG2 hepatoma cells formed a considerable amount of insoluble cytoplasmic inclusions consisting of ubiquitinated proteins and p62 ( Fig. 1a–c ). PA-induced accumulation of protein inclusions had a proportional correlation with both dose ( Supplementary Fig. 1 ) and time ( Supplementary Fig. 2a ); correspondingly, when treated for a longer period (48 h), even a very low dose of PA (50 μM) was able to induce substantial protein inclusions ( Supplementary Fig. 1b ). Although prolonged treatment of high-dose PA (24 and 48 h, 500 μM) provoked apoptosis, there was no significant cell death at 9 h of PA treatment ( Supplementary Fig. 3 ), a time point at which we observed the greatest amount of prominent protein inclusions ( Fig. 1a–c ; Supplementary Fig. 2a ). The inclusions were frequently associated with condensed fibres of keratin ( Supplementary Fig. 4a ) or tubulin ( Supplementary Fig. 4b ) as observed previously for various protein aggregates [28] , [30] . It is interesting to note that the protein aggregates were located away from the ER structure ( Supplementary Fig. 4c ) in which many unfolded proteins typically accumulate during lipotoxicity and obesity [13] . Although another SFA stearic acid (SA) was also able to induce accumulation of p62 ( Supplementary Fig. 2b ), UFA such as oleic acid (OA) and docosahexaenoic acid (DHA) failed to induce such accumulation ( Supplementary Fig. 2c,d ) and actually suppressed the effect of SFA ( Supplementary Fig. 2e,f ). 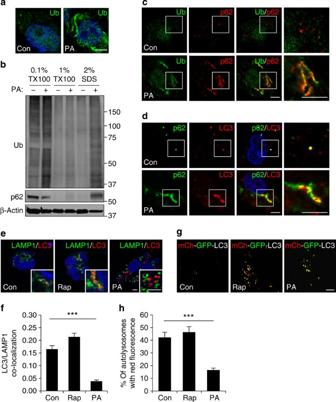Figure 1: SFA induces protein inclusions and arrests autophagy. (a–f) HepG2 cells were treated with bovine serum albumin (Con), 500 μM PA or 100 nM rapamycin (Rap) for 9 h and subjected to following analyses. (a,c–f) Cells were stained with ubiquitin (Ub), p62, LC3 and LAMP1 antibodies and DAPI (blue). Boxed areas are magnified in right-most panels (c,d). Co-localization between LAMP1 and LC3 staining (e) was quantified (f;n=3). (b) Cells were subjected to serial protein extraction (solubility fractionation) with indicated concentration of Triton X-100 (TX100) or sodium dodecyl sulphate (SDS) and analysed by immunoblotting with indicated antibodies. (g,h) HepG2 cells stably transduced with mCherry (mCh)-GFP-LC3-expressing retroviruses were treated with Con, Rap or PA for 9 h and examined under a live confocal microscope (g). Yellow dots represent autophagosomes while red dots indicate autolysosomes in which GFP signal was faded out. Number of autolysosomes was quantified (h;n=7). Scale bar, 5 μm. All data are shown as mean±s.e.m. ***P<0.001 (Student’st-test). Molecular weight markers are indicated in kDa. Figure 1: SFA induces protein inclusions and arrests autophagy. ( a – f ) HepG2 cells were treated with bovine serum albumin (Con), 500 μM PA or 100 nM rapamycin (Rap) for 9 h and subjected to following analyses. ( a , c – f ) Cells were stained with ubiquitin (Ub), p62, LC3 and LAMP1 antibodies and DAPI (blue). Boxed areas are magnified in right-most panels ( c , d ). Co-localization between LAMP1 and LC3 staining ( e ) was quantified ( f ; n =3). ( b ) Cells were subjected to serial protein extraction (solubility fractionation) with indicated concentration of Triton X-100 (TX100) or sodium dodecyl sulphate (SDS) and analysed by immunoblotting with indicated antibodies. ( g , h ) HepG2 cells stably transduced with mCherry (mCh)-GFP-LC3-expressing retroviruses were treated with Con, Rap or PA for 9 h and examined under a live confocal microscope ( g ). Yellow dots represent autophagosomes while red dots indicate autolysosomes in which GFP signal was faded out. Number of autolysosomes was quantified ( h ; n =7). Scale bar, 5 μm. All data are shown as mean±s.e.m. *** P <0.001 (Student’s t -test). Molecular weight markers are indicated in kDa. Full size image SFA induces accumulation of autophagosomes Because defective autophagy can explain excessive accumulation of p62 and ubiquitinated proteins [31] , we examined the level of autophagosomes in cells with an autophagosome marker LC3 (ref. 32 ). During autophagosome formation, LC3 precursor (LC3-I) is proteolytically cleaved and lipidated for incorporation into an autophagosomal membrane as LC3-II. SFA, but not UFA, induced prominent accumulation of autophagosomes as manifested by increased LC3-II levels ( Supplementary Fig. 2a–f ). The patterns of LC3-II expression directly correlated with the patterns of p62 levels ( Supplementary Fig. 2a–f ), and LC3-positive autophagosomes were frequently co-localized with p62 inclusions in SFA-treated cells ( Fig. 1d ). SFA inhibits fusion between autophagosomes and lysosomes To determine whether SFA induces autophagosome accumulation through increased formation or decreased degradation of autophagosomes, we examined autophagy flux in SFA-treated cells through three independent assays [32] . For all assays, cells treated with an autophagy inducer rapamycin were used as a positive control. In the first assay, we incubated cells with bafilomycin, which halts autophagosome degradation by disrupting lysosomal pH homeostasis, and examined the amount of newly formed autophagosomes through LC3-II immunoblotting. As expected, control cells (both untreated and rapamycin-treated cells) showed significantly increased LC3-II levels after bafilomycin application ( Supplementary Fig. 2g,h ). In contrast, PA-treated cells did not exhibit any increase in LC3-II level following bafilomycin addition ( Supplementary Fig. 2g,h ), suggesting that decreased degradation, rather than increased formation, is the cause of PA-induced autophagosome accumulation. The second assay involved staining PA-treated cells with anti-LC3-II and anti-LAMP1 antibodies to visualize autophagosomes and lysosomes, respectively. Although there was a considerable level of association between autophagosomes and lysosomes in control cells, such association was hardly observed in PA-treated cells ( Fig. 1e,f ). We finally utilized an autophagy flux indicator mCherry-GFP-LC3 in the third assay. mCherry-GFP-LC3 initially fluoresces both red and green as it labels autophagosomes. On fusion with lysosomes that exposes mCherry-GFP fluorophore to acidic environment, GFP is denatured and loses its green colour while mCherry maintains its red fluorescence. Thus, all autolysosomes fluoresce only red once the fusion is complete. Although control cells exhibited both autophagosomes and autolysosomes, autolysosomes were very scarce in PA-treated cells ( Fig. 1g,h ). These results collectively indicate that SFA inhibits autophagic flux mainly by blocking the fusion between autophagosomes and lysosomes. Stress pathways do not mediate autophagy arrest on SFA We then tried to determine how SFA can cause a defect in autophagic flux and induce protein inclusion. Several potential physiological consequences of SFA treatment include ceramide accumulation [33] , oxidative stress [34] , ER stress [35] and JNK signalling activation [12] . However, these are signals known to stimulate, rather than inhibit, the autophagic flux in various systems [36] , [37] , [38] , suggesting that these stress pathways may be irrelevant to the effect of SFA on autophagy. To test this, we inhibited ceramide biosynthesis by L -cycloserine and fumonisin B1 ( Supplementary Fig. 5a ), suppressed oxidative stress by butylated hydroxyanisole (BHA) and N -acetylcysteine (NAC; Supplementary Fig. 5b ), reduced ER stress by a chemical chaperone tauroursodeoxycholic acid (TUDCA; Supplementary Fig. 5c ) and inhibited JNK by SP600125 ( Supplementary Fig. 5d ). We also inhibited three ER stress sensor molecules, pancreatic ER kinase (PERK; Supplementary Fig. 5e ), inositol-requiring enzyme 1 alpha (IRE1α; Supplementary Fig. 5f ) and activating transcription factor 6 (ATF6; Supplementary Fig. 5g ) through lentiviruses expressing small hairpin RNA (shRNA) or dominant-negative mutants targeting these molecules. As expected, none of these interventions significantly suppressed the accumulation of p62 and autophagosomes by SFA ( Supplementary Fig. 5 ), suggesting that these signals do not mediate SFA-induced autophagy arrest. SFA induces protein inclusions by inhibiting SERCA We became aware of several recent reports that Tg, an inhibitor of SERCA and inducer of ER stress, could inhibit fusion between autophagosomes and lysosomes [14] , [15] . Because SFA is also known to inhibit SERCA by decreasing ER membrane fluidity [13] , we postulated that SERCA inhibition may provide a common basis for the autophagic arrest induced by Tg and SFA. Confirming the aforementioned reports [14] , [15] , Tg, as well as other SERCA inhibitors such as 2,5- t -butylhydroquinone (TBHQ) and cyclopiazonic acid (CPA), inhibited the association between autophagosomes and lysosomes ( Supplementary Fig. 6a ), arrested autophagic flux ( Supplementary Fig. 6b,c ) and induced accumulation of p62 and LC3-II ( Supplementary Fig. 6d–f ), in the same way as SFA ( Fig. 1 ; Supplementary Fig. 2 ). However, tunicamycin (Tm), an ER stress inducer unrelated to SERCA, did not interfere with autophagic flux ( Supplementary Fig. 6b,c ) and actually decreased p62 levels ( Supplementary Fig. 6d,e,g ), supporting the idea that SERCA inhibition, rather than ER stress induction, is the cause of SFA- and Tg-induced autophagy arrest and protein inclusion formation. shRNA-mediated silencing of SERCA2 also provoked p62 accumulation ( Supplementary Fig. 6h ), while overexpression of SERCA2, which can overcome the obesity-mediated SERCA inhibition [39] , [40] , was able to prevent SFA-induced formation of p62/ubiquitinated protein aggregates ( Supplementary Fig. 6i,j ). These data all strongly indicate that SFA-dependent inhibition of SERCA is the cause of autophagy inhibition and the resulting protein inclusion formation. SFA does not alter lysosomal calcium or proton levels Because both endogenous and overexpressed SERCA proteins were absent from lysosomal or autophagosomal membranes ( Supplementary Fig. 7a,b ), it is not likely that SERCA controls luminal calcium homeostasis in either organelle. Luminal calcium or proton levels of lysosomes, which are important for the autophagosome–lysosome fusion process [41] , were indeed unaffected by SERCA inhibition after SFA or Tg treatment ( Supplementary Fig. 7c,d ). SFA arrests autophagy through elevating cytosolic calcium SFA-mediated elevation in cytosolic calcium level due to prolonged SERCA inhibition ( Fig. 2a–d ) [13] may be the cause of the SFA-induced autophagy defect. This increase in calcium level was substantially averted by application of verapamil and nicardipine, two structurally unrelated calcium channel blockers that prevent leakage of extracellular calcium into cytoplasm ( Fig. 2a–d ). To our surprise, application of verapamil and nicardipine strongly reduced SFA-induced accumulation of p62 and ubiquitinated proteins in the insoluble compartments of cells ( Fig. 2e–h ). Immunofluorescence microscopy confirmed that the calcium channel blockers very effectively prevented SFA-induced formation of p62 and ubiquitinated protein inclusions ( Fig. 2i,j ). The calcium channel blockers also restored the association between autophagosomes and lysosomes in SFA-treated cells ( Fig. 2k,l ). Taken together, these results indicate that chronic elevation of cytosolic calcium level, which can be averted by calcium channel blockers, is primarily responsible for SFA-induced autophagy arrest and protein inclusion formation. 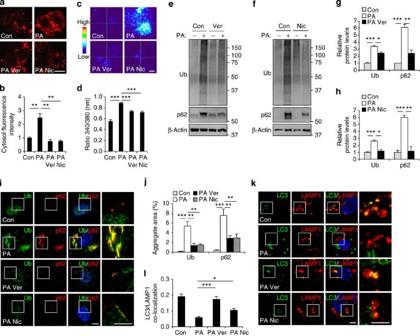Figure 2: Calcium channel blockers suppress SFA-induced protein inclusion formation. HepG2 cells were treated with bovine serum albumin (Con or (−)), PA (500 μM), PA+verapamil (Ver, 50 μM) or PA+nicardipine (Nic, 100 μM) for 9 h. (a–d) After each treatment, cells were loaded with a calcium indicator X-Rhod-1-AM (a,b) or Fura-2-AM (c,d). Calcium levels were visualized by laser confocal microscopy (a) or by dual fluorescent microscopy (c, 340/380 nm ratio image) and quantified (b,d;n=8 and 30, respectively). (e–h) Cells with indicated treatments were subjected to solubility fractionation. 1% Triton X-100-insoluble fractions were dissolved in 2% SDS, analysed by immunoblotting (e,f) and quantified (g,h;n=3). (i–l) Cells with indicated treatments were subjected to immunostaining with indicated antibodies (i,k). DNA was stained with DAPI (blue). Amount of aggregated proteins was quantified (j;n=10). Co-localization between LAMP1 and LC3 was quantified (l;n=4). Boxed areas in fluorescence images are magnified in right-most panels (i,k). Scale bar, 10 μm (a), 20 μm (c), 5 μm (i,k). All data are shown as mean±s.e.m. *P<0.05, **P<0.01, ***P<0.001 (Student’st-test). Molecular weight markers are indicated in kDa. Figure 2: Calcium channel blockers suppress SFA-induced protein inclusion formation. HepG2 cells were treated with bovine serum albumin (Con or (−)), PA (500 μM), PA+verapamil (Ver, 50 μM) or PA+nicardipine (Nic, 100 μM) for 9 h. ( a – d ) After each treatment, cells were loaded with a calcium indicator X-Rhod-1-AM ( a , b ) or Fura-2-AM ( c , d ). Calcium levels were visualized by laser confocal microscopy ( a ) or by dual fluorescent microscopy ( c , 340/380 nm ratio image) and quantified ( b , d ; n =8 and 30, respectively). ( e – h ) Cells with indicated treatments were subjected to solubility fractionation. 1% Triton X-100-insoluble fractions were dissolved in 2% SDS, analysed by immunoblotting ( e , f ) and quantified ( g , h ; n =3). ( i – l ) Cells with indicated treatments were subjected to immunostaining with indicated antibodies ( i , k ). DNA was stained with DAPI (blue). Amount of aggregated proteins was quantified ( j ; n =10). Co-localization between LAMP1 and LC3 was quantified ( l ; n =4). Boxed areas in fluorescence images are magnified in right-most panels ( i , k ). Scale bar, 10 μm ( a ), 20 μm ( c ), 5 μm ( i , k ). All data are shown as mean±s.e.m. * P <0.05, ** P <0.01, *** P <0.001 (Student’s t -test). Molecular weight markers are indicated in kDa. Full size image Calcium channels are expressed in liver cells Many voltage-dependent calcium channels, the targets of verapamil and nicardipine, are expressed in both HepG2 cells and mouse liver ( Supplementary Fig. 8a–e ) [42] . shRNA-mediated silencing of α1 D /Ca v 1.3, the most highly expressed calcium channel isoform in HepG2 cells ( Supplementary Fig. 8d ) [42] , significantly decreased p62 protein inclusion in SFA-treated cells ( Supplementary Fig. 8e,f ), although the decrease in ubiquitinated protein inclusion was not as apparent. The incompleteness in restoration suggests that α1 C /Ca v 1.2 or other unknown calcium channels may have contributed to the hepatocyte calcium influx during SFA treatment. Prolonged calcium influx induces protein inclusions Glucagon, phenylephrine and vasopressin, which can elevate cytosolic calcium level in hepatocytes through activation of inositol trisphosphate receptor [43] , were able to induce protein inclusions ( Supplementary Fig. 9a ), although the extent of this induction was substantially less than those due to high-dose SFA (500 μM). In contrast, ryanodine receptor agonists, which can elevate cytosolic calcium concentration in muscles and neurons, had minimal effects on protein inclusions ( Supplementary Fig. 9b ) most likely because ryanodine receptors are not expressed in liver cells [44] , [45] , or even if expressed, they play a relatively minor role [46] . Verapamil suppresses hepatosteatosis Because of the dramatic effect calcium channel blockers had in restoring autophagy flux in vitro ( Fig. 2 ), we proceeded to use a mouse model of obesity to determine whether they could be a viable therapeutic option for obesity-associated autophagy defects and associated pathologies. Ten days of verapamil administration slightly reduced body weight of high-fat diet (HFD)-kept obese mice ( Fig. 3a ) without any substantial change in food consumption rates ( Fig. 3b ). Although livers from control mice under HFD displayed pink colour due to fat accumulation (hepatosteatosis), the colour of livers from verapamil-administered mice was normal red ( Fig. 3c ). The liver mass was also significantly reduced by verapamil administration ( Fig. 3d ), while the weight of epididymal white adipose tissue remained the same ( Fig. 3e ). Although verapamil exerted minimal effects on the expression of adipokines and adipocytokines in epididymal white adipose tissue ( Fig. 3f–h ), hematoxylin and eosin staining and Oil Red O staining confirmed that verapamil reduced HFD-induced accumulation of hepatic lipid droplets ( Fig. 3i,j ). 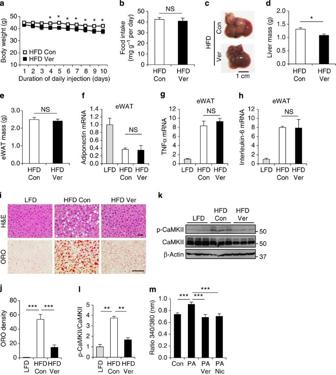Figure 3: Verapamil relieves hepatosteatosis of obese mice. Four-month-old C57BL/6 male mice kept on HFD for 2 months were subjected to daily administration of phosphate-buffered saline (Con,n=4) or verapamil (Ver, 25 mg per kg body weight, i.p.,n=3) for 10 days. Low-fat diet (LFD)-kept mice (n=5) of same age were used as a negative control. (a) Body weight was daily monitored during injection period. (b) Daily food consumption was measured during injection period. (c) Livers were collected from indicated mice and photographed. (d,e) Total liver mass (d) and total epididymal white adipose tissue (eWAT) mass (e) were measured from indicated mice. (f–h) Relative mRNA expression was analysed from eWAT of indicated mice through quantitative reverse transcription–PCR. (i,j) Liver sections were analysed by hematoxylin and eosin (H&E, upper panels) and Oil Red O (ORO, lower panels) staining (i). ORO densities were quantified (j). (k,l) Calcium-induced CaMKII autophosphorylation in livers was analysed by immunoblotting (k) and quantified (l). (m) Primary hepatocytes from 2-month-old C57BL/6 mice kept on LFD were treated with bovine serum albumin (Con), PA (500 μM), PA+verapamil (Ver, 50 μM) or PA+nicardipine (Nic, 100 μM) for 12 h. After each treatment, cells were loaded with a calcium indicator Fura-2-AM. Calcium levels were visualized by dual fluorescent microscopy at 340/380 nm, and ratio of fluorescence intensities of Fura-2-AM at 340 nm over 380 nm was quantified (n=17). Scale bar, 1 cm (c), 200 μm (i). All data are shown as mean±s.e.m. *P<0.05, **P<0.01, ***P<0.001 (Student’st-test). Molecular weight markers are indicated in kDa. Figure 3: Verapamil relieves hepatosteatosis of obese mice. Four-month-old C57BL/6 male mice kept on HFD for 2 months were subjected to daily administration of phosphate-buffered saline (Con, n =4) or verapamil (Ver, 25 mg per kg body weight, i.p., n =3) for 10 days. Low-fat diet (LFD)-kept mice ( n =5) of same age were used as a negative control. ( a ) Body weight was daily monitored during injection period. ( b ) Daily food consumption was measured during injection period. ( c ) Livers were collected from indicated mice and photographed. ( d , e ) Total liver mass ( d ) and total epididymal white adipose tissue (eWAT) mass ( e ) were measured from indicated mice. ( f – h ) Relative mRNA expression was analysed from eWAT of indicated mice through quantitative reverse transcription–PCR. ( i , j ) Liver sections were analysed by hematoxylin and eosin (H&E, upper panels) and Oil Red O (ORO, lower panels) staining ( i ). ORO densities were quantified ( j ). ( k , l ) Calcium-induced CaMKII autophosphorylation in livers was analysed by immunoblotting ( k ) and quantified ( l ). ( m ) Primary hepatocytes from 2-month-old C57BL/6 mice kept on LFD were treated with bovine serum albumin (Con), PA (500 μM), PA+verapamil (Ver, 50 μM) or PA+nicardipine (Nic, 100 μM) for 12 h. After each treatment, cells were loaded with a calcium indicator Fura-2-AM. Calcium levels were visualized by dual fluorescent microscopy at 340/380 nm, and ratio of fluorescence intensities of Fura-2-AM at 340 nm over 380 nm was quantified ( n =17). Scale bar, 1 cm ( c ), 200 μm ( i ). All data are shown as mean±s.e.m. * P <0.05, ** P <0.01, *** P <0.001 (Student’s t -test). Molecular weight markers are indicated in kDa. Full size image Verapamil reduces obesity-induced cytosolic calcium in liver We confirmed that verapamil modulated calcium homeostasis in mouse hepatocytes; HFD-induced autophosphorylation of calcium/calmodulin-dependent protein kinase II (CaMKII) [47] , [48] , which is indicative of an elevated level of cytosolic calcium in hepatocytes [49] , was strongly suppressed by verapamil administration ( Fig. 3k,l ). PA-induced elevation of cytosolic calcium level in primary mouse hepatocytes was also suppressed by verapamil ( Fig. 3m ). Verapamil restores autophagic flux in liver of obese mice We examined the level of protein inclusion formation in obese mouse liver. As formerly reported [29] , [50] , obesity induced prominent accumulation of p62 and ubiquitinated proteins in insoluble fractions of liver lysates ( Fig. 4a–d ). The protein inclusions, however, almost completely disappeared after administration of verapamil ( Fig. 4a–d ), demonstrating that verapamil is capable of resolving HFD-induced accumulation of both lipid droplets and protein inclusions. Immunohistochemistry of p62 in mouse liver also confirmed that verapamil administration is sufficient to eliminate p62-containing protein inclusions induced by obesity ( Fig. 4e,f ). As observed in SFA-treated HepG2 cells, HFD induced accumulation of insoluble LC3-II ( Fig. 5a,b ), most likely as a result of fusion defects between autophagosomes and lysosomes. Indeed, obesity substantially decreased the association between autophagosomes and lysosomes in mouse liver ( Fig. 5c,d ) in consistence with previous reports [6] , [22] . Verapamil administration allowed autophagosomes and lysosomes to re-associate ( Fig. 5c,d ) and subsequently suppressed accumulation of LC3-II in obese mouse liver ( Fig. 5a,b ). Thus, as observed in cultured cells, calcium channel blockers can restore the fusion between autophagosomes and lysosomes and subsequently autophagic removal of protein inclusions and lipid droplets in vivo . 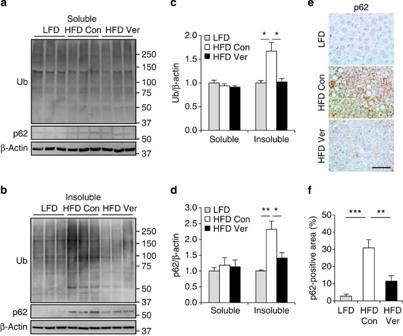Figure 4: Verapamil suppresses obesity-induced accumulation of protein aggregates. Four-month-old C57BL/6 male mice kept on HFD for 2 months were subjected to daily administration of phosphate-buffered saline (Con,n=4) or verapamil (Ver, 25 mg per kg body weight, i.p.,n=3) for 10 days. Low-fat diet-kept mice (n=5) of same age were used as a negative control. (a–d) Livers were subjected to solubility fractionation. 1% Triton X-100-soluble (a) and -insoluble (b) fractions were analysed by immunoblotting (a,b) and quantified (c,d). (e,f) Paraffin sections of indicated livers were subjected to p62 immunostaining and hematoxylin counterstaining (e). p62-positive areas were quantified (f). Scale bar, 200 μm (e). All data are shown as mean±s.e.m. *P<0.05, **P<0.01, ***P<0.001 (Student’st-test). Molecular weight markers are indicated in kDa. Figure 4: Verapamil suppresses obesity-induced accumulation of protein aggregates. Four-month-old C57BL/6 male mice kept on HFD for 2 months were subjected to daily administration of phosphate-buffered saline (Con, n =4) or verapamil (Ver, 25 mg per kg body weight, i.p., n =3) for 10 days. Low-fat diet-kept mice ( n =5) of same age were used as a negative control. ( a – d ) Livers were subjected to solubility fractionation. 1% Triton X-100-soluble ( a ) and -insoluble ( b ) fractions were analysed by immunoblotting ( a , b ) and quantified ( c , d ). ( e , f ) Paraffin sections of indicated livers were subjected to p62 immunostaining and hematoxylin counterstaining ( e ). p62-positive areas were quantified ( f ). Scale bar, 200 μm ( e ). All data are shown as mean±s.e.m. * P <0.05, ** P <0.01, *** P <0.001 (Student’s t -test). Molecular weight markers are indicated in kDa. 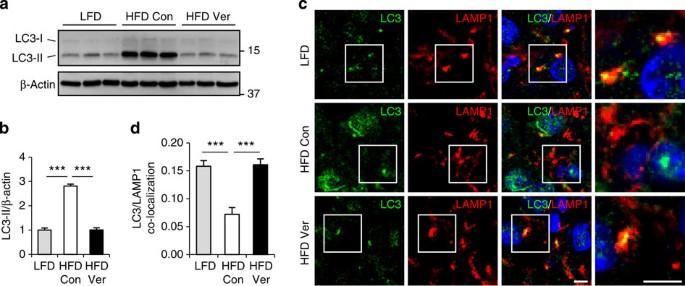Figure 5: Verapamil restores lysosomal degradation of autophagosomes in liver of obese mice. Four-month-old C57BL/6 male mice kept on HFD for 2 months were subjected to daily administration of phosphate-buffered saline (Con,n=4) or verapamil (Ver, 25 mg per kg body weight, i.p.,n=3) for 10 days. Low-fat diet-kept mice (n=5) of same age were used as a negative control. (a,b) Levels of LC3-II from 1% Triton X-100-insoluble fraction of livers were analysed by immunoblotting (a) and quantified (b). (c,d) Frozen sections of indicated livers were subjected to LC3/LAMP1 immunostaining and DAPI counterstaining (c). Co-localization between LC3 and LAMP1 was quantified (d). Boxed areas in fluorescence images are magnified in right-most panels (c). Scale bar, 5 μm (c). All data are shown as mean±s.e.m. ***P<0.001 (Student’st-test). Molecular weight markers are indicated in kDa. Full size image Figure 5: Verapamil restores lysosomal degradation of autophagosomes in liver of obese mice. Four-month-old C57BL/6 male mice kept on HFD for 2 months were subjected to daily administration of phosphate-buffered saline (Con, n =4) or verapamil (Ver, 25 mg per kg body weight, i.p., n =3) for 10 days. Low-fat diet-kept mice ( n =5) of same age were used as a negative control. ( a , b ) Levels of LC3-II from 1% Triton X-100-insoluble fraction of livers were analysed by immunoblotting ( a ) and quantified ( b ). ( c , d ) Frozen sections of indicated livers were subjected to LC3/LAMP1 immunostaining and DAPI counterstaining ( c ). Co-localization between LC3 and LAMP1 was quantified ( d ). Boxed areas in fluorescence images are magnified in right-most panels ( c ). Scale bar, 5 μm ( c ). All data are shown as mean±s.e.m. *** P <0.001 (Student’s t -test). Molecular weight markers are indicated in kDa. Full size image Verapamil suppresses ER stress in liver of obese mice Because autophagy is important for suppressing ER stress [29] , we examined whether verapamil-mediated resumption of autophagy could suppress ER stress in liver of obese mice. Phosphorylation of eukaryotic translation initiation factor 2-alpha (eIF2α) and induction of binding immunoglobulin protein expression, which are ER stress signalling markers elevated in mouse liver on HFD-induced obesity [51] , were both strongly suppressed by verapamil administration ( Supplementary Fig. 10a–c ). Verapamil suppresses steatohepatitis Liver inflammation, characterized by increased macrophage infiltration into the liver, is a hallmark of NASH pathologies in addition to accumulation of lipid droplets and protein inclusions [52] . Because liver inflammation can be provoked by either HFD-induced obesity [53] or genetic inhibition of autophagy [26] , [54] , we were interested in the effect that calcium channel blockers may have on resolving obesity-associated liver inflammation. Verapamil administration was found to reduce liver inflammation in livers from HFD-kept obese mice, as manifested by decreased macrophage number that is comparable to that of low-fat diet-kept lean mice ( Fig. 6a,b ). These results add more evidence that calcium channel blockers can have a potential as therapeutics for NASH pathologies. 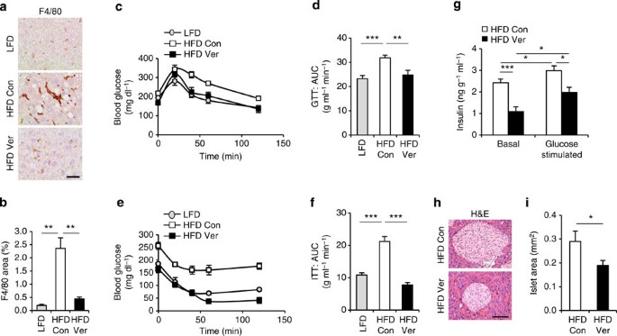Figure 6: Verapamil reduces liver inflammation and improves metabolic homeostasis. Four-month-old C57BL/6 male mice kept on HFD for 2 months were subjected to daily administration of phosphate-buffered saline (Con,n=4) or verapamil (Ver, 25 mg per kg body weight, i.p.,n=3) for 10 days. Low-fat diet-kept mice of same age (n=5) were used as a negative control. (a,b) Liver sections were subjected to F4/80 immunostaining, which visualizes macrophage infiltration and hematoxylin counterstaining (a). F4/80-positive areas were quantified (b). (c–f) Glucose tolerance tests (GTT,c,d) and insulin tolerance tests (ITT,e,f) were conducted using indicated mice (c,e). Area under the curve (AUC) was quantified from GTT and ITT data (d,f). (g) Serum insulin levels were measured from indicated mice before (Basal) and 10 min after (Glucose stimulated) glucose injection (n=4). (h,i) Pancreas sections were analysed by hematoxylin and eosin (H&E) staining (h). Islet areas were quantified (i;n=4). Scale bar, 200 μm (a), 100 μm (h). All data are shown as mean±s.e.m. *P<0.05, **P<0.01, ***P<0.001 (Student’st-test). Figure 6: Verapamil reduces liver inflammation and improves metabolic homeostasis. Four-month-old C57BL/6 male mice kept on HFD for 2 months were subjected to daily administration of phosphate-buffered saline (Con, n =4) or verapamil (Ver, 25 mg per kg body weight, i.p., n =3) for 10 days. Low-fat diet-kept mice of same age ( n =5) were used as a negative control. ( a , b ) Liver sections were subjected to F4/80 immunostaining, which visualizes macrophage infiltration and hematoxylin counterstaining ( a ). F4/80-positive areas were quantified ( b ). ( c – f ) Glucose tolerance tests (GTT, c , d ) and insulin tolerance tests (ITT, e , f ) were conducted using indicated mice ( c , e ). Area under the curve (AUC) was quantified from GTT and ITT data ( d , f ). ( g ) Serum insulin levels were measured from indicated mice before (Basal) and 10 min after (Glucose stimulated) glucose injection ( n =4). ( h , i ) Pancreas sections were analysed by hematoxylin and eosin (H&E) staining ( h ). Islet areas were quantified ( i ; n =4). Scale bar, 200 μm ( a ), 100 μm ( h ). All data are shown as mean±s.e.m. * P <0.05, ** P <0.01, *** P <0.001 (Student’s t -test). Full size image Verapamil suppresses obesity-induced insulin resistance In addition to being responsible for accumulation of lipid droplets and protein inclusions [6] , [26] , [31] , autophagy defects and NASH can both promote the development of insulin resistance [29] , [52] , the infamous precursor of type 2 diabetes. Thus, we questioned whether calcium channel blockers could be used for correcting insulin resistance in HFD-kept obese mice. HFD-induced obesity provoked glucose intolerance ( Fig. 6c,d ) and insulin resistance ( Fig. 6e,f ) in mice as formerly reported [55] . Intriguingly, verapamil administration strongly suppressed both metabolic pathologies; glucose intolerance ( Fig. 6c,d ) and insulin resistance ( Fig. 6e,f ) were restored back to the normal level by verapamil administration. Serum insulin level ( Fig. 6g ) and pancreatic islet size ( Fig. 6h,i ) were significantly decreased by verapamil administration, indicating that obesity-associated hyperinsulinemia [56] was also suppressed. These results suggest that calcium channel blockers can be effective for correction of insulin resistance and blood glucose homeostasis defects during obesity. Verapamil improves cardiac functionality in obese mice Finally, we tested the effect of verapamil on blood pressure and cardiac functionality, which are partially controlled by voltage-dependent calcium channels. Verapamil administration induced only a slight decrease in blood pressure of HFD-kept obese mice, which was not enough to reach the level of statistical significance ( Fig. 7a ). We also did not observe substantial changes in heart size; left ventricular (LV) wall mass ( Fig. 7b ) and diastolic LV volume ( Fig. 7c ) remained similar between verapamil-treated and -untreated groups. Intriguingly, there was a significant reduction in systolic LV volume ( Fig. 7d ) and an increase in LV ejection fraction (% EF; Fig. 7e ), suggesting that heart contractility may have been improved by verapamil treatment. However, verapamil-induced elevation of LV stroke volume and cardiac output was not statistically significant ( Fig. 7f,g ). 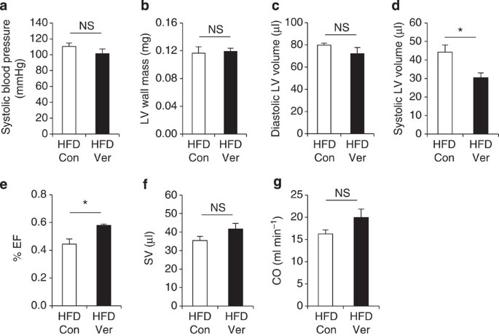Figure 7: Effects of verapamil on blood pressure and cardiac functionality of obese mice. (a–g) Four-month-old C57BL/6 male mice kept on HFD for 2 months were subjected to daily administration of phosphate-buffered saline (Con,n=4) or verapamil (Ver, 25 mg per kg body weight, i.p.,n=4) for 10 days. Systolic blood pressure (a), LV wall mass (b), diastolic LV volume (c), systolic LV volume (d), ejection fraction (e, % EF), stroke volume (f, SV) and cardiac output (g, CO) were analysed by tail-cuff method (a) or echocardiography (b–g). All data are shown as mean±s.e.m. *P<0.05 (Student’st-test). Figure 7: Effects of verapamil on blood pressure and cardiac functionality of obese mice. ( a – g ) Four-month-old C57BL/6 male mice kept on HFD for 2 months were subjected to daily administration of phosphate-buffered saline (Con, n =4) or verapamil (Ver, 25 mg per kg body weight, i.p., n =4) for 10 days. Systolic blood pressure ( a ), LV wall mass ( b ), diastolic LV volume ( c ), systolic LV volume ( d ), ejection fraction ( e , % EF), stroke volume ( f , SV) and cardiac output ( g , CO) were analysed by tail-cuff method ( a ) or echocardiography ( b – g ). All data are shown as mean±s.e.m. * P <0.05 (Student’s t -test). Full size image The autophagy signalling pathway has been extensively studied in the context of hypernutrition and obesity in recent years, and there is now a general consensus that autophagy deregulation contributes to the pathogenesis of diverse obesity-associated metabolic disorders [7] , [20] , [22] , [29] , [57] , [58] , [59] , [60] . However, as the molecular mechanism of obesity interference in autophagy has been obscure, we have not yet been able to develop effective therapeutic strategies for correcting autophagy defects in obese individuals. Our current report suggests that lipotoxicity-induced elevation of cytosolic calcium is primarily responsible for the autophagy defects observed during obesity. Chronic increase in cytosolic calcium level specifically inhibits the fusion between autophagosomes and lysosomes, thereby attenuating the autophagic flux. This attenuation leads to prominent accumulation of undegraded autophagy substrates such as ubiquitinated proteins, p62 aggregates and lipid droplets, ultimately resulting in excessive fat accumulation, ER stress, liver inflammation and insulin resistance. As calcium channel blockers can prevent the cytosolic calcium influx, they have high potential as therapeutic candidates for correcting obesity-induced autophagy defects and preventing their pathological consequences. Indeed, both non-dihydropyridine (verapamil) and dihydropyridine (nicardipine) calcium channel blockers were effective in restoring the autophagic flux and suppressing protein inclusion formation during lipotoxicity. Various calcium channel blockers have been on the pharmaceutical market for around 30 years, and there have been many clinical/pre-clinical studies on their effect on metabolism. To identify specific papers on this subject, we have utilized a computerized natural language processing/text mining tool to screen all the abstracts published in the MEDLINE database [61] . Using this method, we were able to identify 39 papers that describe the causal relationship between calcium channel blockers and metabolic homeostasis in humans or animals. Among them, 25 papers, including several very recent ones [62] , [63] , indicate that calcium channel blockers can improve glucose metabolism and/or liver homeostasis ( Supplementary Table 1a ), which is consistent with our current findings. Many of these papers examine animals or humans associated with either obesity or type 2 diabetes, and these subjects are likely to have obesity/lipotoxicity-associated autophagy defects, which are correctable by calcium channel blockers. In contrast, 14 papers were identified to indicate neutral or even negative effects of calcium channel blockers on metabolism ( Supplementary Table 1b ). Specifically, one large meta-analysis of long-term clinical trials demonstrates that calcium channel blockers are not effective in preventing incidental diabetes in hypertensive patients [64] . However, we should take into account that, even though autophagy is important for prevention of metabolic pathologies and diabetes [29] , autophagic defects, which are correctable by calcium channel blockers, may not be the only cause for diabetes. Thus, it is feasible that calcium channel blocker-mediated restoration of the autophagic flux could not prevent the occurrence of incidental diabetes in certain cases, as they may have arisen from causes other than autophagy misregulation. Nevertheless, our study does suggest that calcium channel blockers have a clinical potential for a subset of patients with NASH and type 2 diabetes whose symptoms are indeed associated with lipotoxicity-induced autophagy arrest. It would therefore be worthwhile to conduct more rigorous human clinical studies focused on the possible usage of calcium channel blockers for NASH and other obesity-associated metabolic pathologies. Antibodies and reagents Ubiquitin (sc-8017), LAMP1 (sc-20011), phospho-PERK (sc-32577), PERK (sc-13073), phospho-c-Jun (sc-822), c-Jun (sc-376488), SERCA2 (sc-376235, sc-8095), ATF6 (sc-22799), eIF2α (sc-11386), CaMKII (sc-5306), α1 C /Ca v 1.2 (sc-16229-R), α1 D /Ca v 1.3 (sc-25687), LC3 (sc-271625) and p62 (sc-28359) antibodies were obtained from Santa Cruz Biotechnology. IRE1α (3294), phospho-CaMKII (12716), phospho-eIF2α (3398), PERK (5683), LC3 (2775), p62 (5114) and calnexin (2679) antibodies were purchased from Cell Signaling Technology. Pan-keratin antibody was obtained from Dr Omary (University of Michigan (UM)) [65] . Actin (JLA20) and tubulin (T5168) antibodies were purchased from Developmental Studies Hybridoma Bank and Sigma, respectively. Fatty acid-free and low-endotoxin bovine serum albumin, PA, SA, OA, DHA, Tm, Tg, BHA, NAC, chlorocresol, L -cycloserine, glucagon, phenylephrine, vasopressin, verapamil and nicardipine were purchased from Sigma. SP600125, bafilomycin and rapamycin were from LC Labs, and fumonisin B1 and suramin were from Cayman Chemical. Cell culture HepG2 cells (gift from Dr Saltiel), a human hepatoma cell line, were cultured in DMEM (Invitrogen) containing 10% fetal bovine serum (Sigma), 50 U ml −1 penicillin and 50 mg ml −1 streptomycin. All cultures were maintained in a 37 °C incubator with 5% CO 2 . De-lipidated low-endotoxin bovine serum albumin was loaded with different fatty acids and applied to cultured cells [12] . Viral procedures The lentiviral plasmid for sh-SERCA2 (Broad Institute TRC Portal accession code TRCN0000038532), sh-PERK (TRCN0000001401 and TRCN0000001399), sh-ATF6 (TRCN0000017853) and sh-α1 D (TRCN0000044693 and TRCN0000044695) was purchased from Open Biosystems (Huntsville, AL). Lentiviral LAMP1-mRFP, Lentiviral IRE1α DN and retroviral mCherry-GFP-LC3 constructs were obtained from Addgene (Cambridge, MA). Adenoviruses expressing the 2b isoform of SERCA (Ad-SERCA2b) were gifts from Dr Hotamisligil [40] . Viruses were generated and amplified in the Vector Core facility at the UM. Solubility fractionation Cells were lysed in a lysis buffer [66] containing 0.1% Triton X-100. Cell and tissue lysates were centrifuged at 15,000 r.p.m. for 15 min at 4 °C to separate pellets from supernatants. Pellets were resuspended in a lysis buffer containing 1% Triton X-100 and then subjected to centrifugation at 15,000 r.p.m. for 15 min at 4 °C. After centrifugation, pellets were resuspended in a lysis buffer containing 2% SDS and boiled in SDS sample buffer. Liver tissues were directly lysed in a lysis buffer containing 1% Triton X-100 and centrifuged at 15,000 r.p.m. for 15 min at 4 °C. Pellets were dissolved in a lysis buffer containing 2% SDS. Supernatants (soluble fraction) and resuspended pellets (insoluble fraction) were boiled in SDS sample buffer. Immunoblotting Unless otherwise noted, cells and tissues were lysed in radioimmunoprecipitation assay buffer (50 mM Tris–HCl, pH 7.4; 150 mM NaCl; 1% deoxycholate Na; 1% NP-40; 0.1% SDS; and complete protease inhibitor cocktail (Roche)). Lysates were centrifuged at 15,000 r.p.m. for 15 min at 4 °C. Lipid layer was removed and supernatant was collected. Protein concentration was measured using Bio-rad protein assay kit. Lysates were boiled in SDS sample buffer for 5 min, separated by SDS–polyacrylamide gel electrophoresis, transferred to polyvinylidene fluoride membranes and probed with primary antibodies (1:200 for Santa Cruz antibodies, and 1:1,000 for Cell Signaling and Developmental Studies Hybridoma Bank antibodies). After incubation with secondary antibodies conjugated with horseradish peroxidase (1:2,000), chemiluminescence was detected using LAS4000 (GE) systems. Uncropped images of immunoblots presented in the main paper are provided in Supplementary Information ( Supplementary Fig. 11 ). Immunocytochemistry and TUNEL analysis Cells grown on coverslips were fixed with 4% paraformaldehyde and incubated overnight with primary antibodies (1:50 for Santa Cruz antibodies, 1:200 for pan-keratin and tubulin antibodies and 1:400 for Cell Signaling antibodies). After washing, cells were incubated with Alexa Fluor-conjugated secondary antibodies (Invitrogen, 1:250) for 1.5 h and counterstained with 4',6-diamidino-2-phenylindole (DAPI; Invitrogen). Apoptotic cells were determined by TUNEL (terminal dUTP nick-end labeling) with In Situ Cell Death Detection Kit-TMR-Red (Roche). Samples were analysed under an epifluorescence-equipped microscope (Meiji) or a laser confocal microscope (Olympus). RNA analysis Total RNA was extracted from tissues or cells using Trizol reagent (Invitrogen), and complementary DNA was made using MMLV-RT (Invitrogen) and random hexamers (Invitrogen). Quantitative reverse transcription–PCR was performed in a Real-Time PCR detection system (Applied Biosystems) with iQ SYBR Green Supermix (Bio-rad) and relevant primers ( Supplementary Table 2 ). Relative mRNA expression was calculated from the comparative threshold cycle ( C t ) values relative to mouse β-actin or human cyclophilin A. To determine human XBP1 splicing, PCR products of spliced (XBP1-s) and unspliced (XBP1-u) XBP1 mRNA were separated by electrophoresis on a 2.5% agarose gel and visualized by ethidium bromide staining. Calcium measurements For lysosomal calcium measurements, we performed Oregon Green 488 BAPTA-1 dextran (OGBD) labelling [41] . In this assay, cells with a stable transduction of LAMP1-mRFP lentiviruses were loaded with 0.1 mg ml −1 OGBD (Invitrogen) for 30 min. For cytosolic calcium measurements, we performed X-Rhod-1 and Fura-2 labelling assays. In these assays, cells were loaded with 1 μM X-Rhod-1-AM (Invitrogen) or 1 μM Fura-2-AM (Invitrogen) for 30 min. For OGBD and X-Rhod-1 imaging, the cells were examined under a temperature- and CO 2 -controlled laser confocal microscope (Olympus); for ratiometric Fura-2 imaging, cells were examined under a temperature- and CO 2 -controlled fluorescence microscope equipped with excitation wavelengths of 340 and 380 nm (Till Polychrome V, Till Photonics, Gräfelfing, Germany), a 410-dLcp beamsplitter, a D510/80 wide-band emission filter (Chroma Technology, Rockingham, VT, USA) and a Quant-EM camera (Photometrics, Tucson, AZ, USA). LysoSensor staining For LysoSensor labelling, cells with stable transduction of LAMP1-mRFP lentiviruses were stained with 1 μM LysoSensor Green DND-189 (Invitrogen) for 30 min. After washing with phosphate-buffered saline, live cells were imaged immediately on a temperature- and CO 2 -controlled laser confocal microscope (Olympus). Mice and diets Mice were maintained in filter-topped cages and were given free access to autoclaved regular chow diet (low-fat diet) or HFD (S3282, Bio-Serv) and water at the UM according to the NIH and institutional guidelines. The strain, sex and age of mice for each experiment are described in the corresponding figure legend section. All animal studies were ethically approved (protocol approval number: PRO00001461) and overseen by the University Committee on Use and Care of Animals at the UM. Glucose and insulin tolerance tests For glucose and insulin tolerance tests, mice were starved for 6 h. Blood was drawn from a tail nick at the indicated time points after i.p. injection of glucose (1 g per kg body weight) or insulin (0.65 U per kg body weight). Blood glucose was instantly measured with OneTouch Ultra glucose meter (Lifescan). Serum insulin levels were measured with an ultrasensitive mouse insulin ELISA kit (Crystal Chem). Mice were tested for insulin resistance at 5 days and glucose tolerance at 7 days after initiation of phosphate-buffered saline and verapamil treatments. Histology Tissues were fixed in 10% formalin or embedded in Tissue-Tek optimum cutting temperature (OCT) compound (Sakura Finetek) for paraffin or frozen block preparation, respectively. Paraffin-embedded tissues were used for hematoxylin and eosin or immunohistochemical staining of p62 (1:50) and F4/80 (1:100). Frozen tissue sections were stained with Oil Red O or immunostained with LC3 (1:400) and LAMP1 (1:50) antibodies. Hematoxylin or DAPI counterstaining was applied to visualize nuclei. Samples were analysed under a light microscope (Meiji) or a laser confocal microscope (Olympus). Primary cell culture Primary mouse hepatocytes were isolated and cultured from livers of 2-month-old lean mice by a two-step collagenase digestion with 100 U ml −1 collagenase in Hank’s Balanced Salt Solution at pH 7.4. After dissection, the liver was placed in DMEM and carefully pulled apart to release hepatocytes. Hepatocytes in DMEM were passed through a 100-μm cell strainer and then spun at 50 g for 1 min. The pellet was resuspended in DMEM and then spun at 50 g for 10 min in a Percoll gradient to remove dead hepatocytes. The viable primary hepatocytes were washed with DMEM at 50 g for 10 min and cultured in 10% fetal bovine serum and DMEM. Echocardiography Induction of anaesthesia was performed in an enclosed container filled with 5% isoflurane. After induction, the mice were placed on a warming pad to maintain body temperature. Isoflurane (1–1.5%) was supplied via a nose cone to maintain a surgical plane of anaesthesia. Hair was removed from the upper abdominal and thoracic area with depilatory cream. Transthoracic echocardiography was performed in the supine or left lateral position. Two-dimensional (2D) and M-mode echocardiographic images were recorded using a Vevo 2100 high-resolution in vivo micro-imaging system (Visual Sonics). We measured LV ejection fraction from the 2D long axis view. In addition, we measured systolic and diastolic dimensions and wall thickness by M-mode in the parasternal short axis view at the level of the papillary muscles. Fractional shortening and ejection fraction were also calculated from the M-mode parasternal short axis view. Noninvasive blood pressure measurement Systolic blood pressure was measured using a BP-2000 noninvasive tail-cuff system (Visitech, Apex, NC) [67] . Quantification and statistics Immunoblot images were quantified by densitometry, and protein expressions were expressed as relative band intensities. Fluorescence images were analysed using ImageJ (NIH) software equipped with Just Another Co-localization Plugin (JACoP). Relative calcium levels were quantified from cells by the cytosolic intensity of X-Rhod-1 fluorescence or by the ratio between Fura-2 intensities at 340 nm and 380 nm. Co-localization of different proteins was expressed as Pearson’s coefficient. Statistical significance of differences between two groups was calculated using a Student’s t -test. P values equal to or above 0.05 were considered not statistically significant (NS). Literature search In addition to the keyword-based literature search, semantic-based text mining was conducted utilizing the previously described algorithm [61] . One hundred and seventy-one texts that imply causal relationships between ‘Amlodipine, Aranidipine, Azelnidipine, Barnidipine, Benidipine, Cilnidipine, Clevidipine, Isradipine, Efonidipine, Felodipine, Lacidipine, Lercanidipine, Manidipine, Nicardipine, Nifedipine, Nilvadipine, Nimodipine, Nisoldipine, Nitrendipine, Pranidipine, Verapamil, Gallopamil, Fendiline, Diltiazem, Mibefradil, Bepridil, Flunarizine, Fluspirilene, Fendiline’ and ‘Glucose, Fat, Lipid, Free fatty acid, Insulin, Hyperglycemia, Diabetes, Hepatosteatosis, Steatohepatitis, Inflammation, Autophagy, Glucose intolerance, Insulin resistance’ were discovered from the MEDLINE abstract database. These pre-screened texts were manually examined to identify papers that describe the metabolic effect of calcium channel blockers in human and animal systems. How to cite this article: Park, H.-W. et al. Pharmacological correction of obesity-induced autophagy arrest using calcium channel blockers. Nat. Commun. 5:4834 doi: 10.1038/ncomms5834 (2014).